NMDA receptor activation requires remodelling of intersubunit contacts within ligand-binding heterodimers Two classes of glutamate-activated channels mediate excitation at central synapses: N -methyl- D -aspartic acid (NMDA) receptors and non-NMDA receptors. Despite substantial structural homology, each class generates signals with characteristic kinetics and mediates distinct synaptic functions. In non-NMDA receptors, the strength of intersubunit contacts within ligand-binding domains is inversely correlated with functional desensitization. Here we test how the strength of these contacts affects NMDA receptor activation by combining mutagenesis and single-channel current analyses. We show that receptors with covalently linked dimers had significantly lower activity due to high barriers to opening and unstable open states but had intact desensitization. On the basis of these observations, we suggest that in NMDA receptors rearrangements at the heterodimer interface represent an early and integral step of the opening sequence but are not required for desensitization. These results demonstrate distinct functional roles in the activation of NMDA and non-NMDA glutamate-gated channels for largely conserved intersubunit contacts. For all glutamate-gated channels, agonist-binding in the cleft formed by two dynamic lobes, D1 and D2, of ligand-binding domains (LBDs) is the event that energizes resting receptors to either open or desensitize [1] , [2] . The present model for glutamate receptor gating postulates that the mechanical tension produced by agonist-induced cleft-closure can be relieved either by pulling on connected pore-lining helices, which results in channel opening, or by disrupting the D1-D1 intersubunit interface within each LBD dimer, which results in channel desensitization [3] , [4] , [5] . Consistent with this model, in alpha-amino-3-hydroxy-5-methyl-4-isoxazole propionate (AMPA)- and kainate- sensitive glutamate receptors, perturbations of D1-D1 contacts that strengthen the dimer interface prevent desensitization, whereas those that weaken it facilitate desensitization [6] , [7] , [8] , [9] , [10] . By analogy, dimer separation is assumed to represent the physical substrate of NMDA receptor desensitization [11] ; however, direct evidence is lacking. To test the functional role of a strong heterodimer interface in NMDA receptor gating we set out to delineate how perturbing this interface affects the activation mechanism of NMDA receptors. Furukawa et al . [12] showed that in the isolated GluN1/GluN2A LBD heterodimer, N521 and L777 of GluN1 are in close proximity with L780 and E516 of GluN2A, respectively, and substituting pairs of cysteine residues at these four positions in full-length GluN1/GluN2A receptors (Mt1/Mt1), results in cell surface receptors that are spontaneously crosslinked but functional, and whose activity is augmented by dithiothreitol (DTT) treatment. A separate study showed that crosslinked Mt1/Mt1 receptors are resistant to allosteric inhibition and become more sensitive than wild-type (Wt) receptors upon DTT treatment, which suggested the possibility that crosslinked receptors cannot desensitize [11] . To more clearly define the role of intersubunit interactions within NMDA receptor LBDs, we examined the activation mechanism of Mt1/Mt1 receptors in oxidizing and reducing conditions. Here we find that stabilizing the LBD dimer with disulphide bridges deeply impair the channel opening reaction but has no effect on desensitization. Conversely, restoring flexibility across the heterodimer interface by reducing the engineered intersubunit bonds allows Mt1/Mt1 receptors to reach open states that have native-like stabilities. On the basis of these results, we propose that the NMDA receptor activation sequence but not its desensitization involves the relative repositioning of subunits within ligand-binding domains and we suggest that the intramolecular interfaces of NMDA and non-NMDA receptors may have distinct functional roles. Crosslinked receptors produce desensitizing currents Consistent with previous studies [11] , [12] , we found that Mt1/Mt1 receptors expressed in HEK 293 cells were functional, their activity was strongly potentiated by DTT treatment, and DTT treatment effectively induced dimer dissociation ( Fig. 1a–c ; Supplementary Fig. S1 ). However, contrary to the presumption that crosslinking prevents desensitization, whole-cell currents desensitized with kinetics comparable to those of wild-type (Wt/Wt) receptors, and reducing agents (DTT 10 mM, 2 min) strongly potentiated current amplitudes and reduced macroscopic desensitization ( Fig. 1b ). These effects were fully reversible along several reducing/oxidizing cycles ( Fig. 1d ), indicating that the majority of receptors reaching the membrane were in oxidized form and that the DTT-induced changes in current amplitude and kinetics resulted from increased flexibility at the dimer interface. 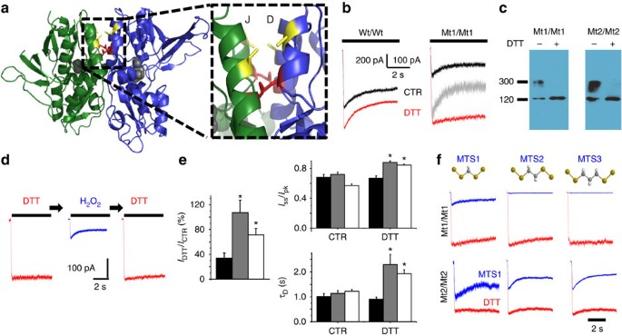Figure 1: Macroscopic properties of Mt1/Mt1 receptors. (a) Crystal structure of the GluN1/GluN2A LBD heterodimer (PDB: 2A5T) illustrates the residues changed to cysteines in this study. Mt1/Mt1 receptors have cysteines (red) at N521 and L777 of GluN1, and E516 and L780 of GluN2A. Mt2/Mt2 has cysteines (yellow) at Q525 and L774 of GluN1 and E520 and L777 of GluN2A. (b) Whole-cell currents recorded from HEK 293 cells expressing Wt/Wt or Mt1/Mt1 receptors in control (CTR, black) and reducing (DTT, red) conditions. CTR normalized to peak of DTT response is in grey. (c) Western blot of proteins solubilized from HEK 293 cells expressing Mt1/Mt1 or Mt2/Mt2 receptors and probed with an anti-GluN1 antibody illustrate a DTT-sensitive, high-molecular-weight band indicative of crosslinked heterodimer formation. (d) Kinetics of Mt1/Mt1 receptors are reversibly modulated by reducing (DTT, red)/oxidizing (hydrogen peroxide, H2O2, blue) treatment cycles. (e) Summary of whole-cell current properties (mean±s.e.m.) for Wt/Wt (black,n=6), Mt1/Mt1 (grey,n=12) and Mt2/Mt2 (white,n=19); asterisk indicatesP<0.05 relative to CTR (Student'st-test). (f) Traces recorded from DTT-treated Mt1/Mt1 or Mt2/Mt2 (red) and after exposure to bifunctional crosslinking reagents (blue). Figure 1: Macroscopic properties of Mt1/Mt1 receptors. ( a ) Crystal structure of the GluN1/GluN2A LBD heterodimer (PDB: 2A5T) illustrates the residues changed to cysteines in this study. Mt1/Mt1 receptors have cysteines (red) at N521 and L777 of GluN1, and E516 and L780 of GluN2A. Mt2/Mt2 has cysteines (yellow) at Q525 and L774 of GluN1 and E520 and L777 of GluN2A. ( b ) Whole-cell currents recorded from HEK 293 cells expressing Wt/Wt or Mt1/Mt1 receptors in control (CTR, black) and reducing (DTT, red) conditions. CTR normalized to peak of DTT response is in grey. ( c ) Western blot of proteins solubilized from HEK 293 cells expressing Mt1/Mt1 or Mt2/Mt2 receptors and probed with an anti-GluN1 antibody illustrate a DTT-sensitive, high-molecular-weight band indicative of crosslinked heterodimer formation. ( d ) Kinetics of Mt1/Mt1 receptors are reversibly modulated by reducing (DTT, red)/oxidizing (hydrogen peroxide, H 2 O 2 , blue) treatment cycles. ( e ) Summary of whole-cell current properties (mean±s.e.m.) for Wt/Wt (black, n =6), Mt1/Mt1 (grey, n =12) and Mt2/Mt2 (white, n =19); asterisk indicates P <0.05 relative to CTR (Student's t -test). ( f ) Traces recorded from DTT-treated Mt1/Mt1 or Mt2/Mt2 (red) and after exposure to bifunctional crosslinking reagents (blue). Full size image To determine whether these effects were specific to the positions used to covalently tether the GluN1 and GluN2A subunits, we tested a second mutant whose dimer interface was reinforced with disulphide bridges between Q525 and L774 of GluN1, and E520 and L777 of GluN2A, respectively (Mt2/Mt2; Fig. 1a ). These residues are located one helix-turn higher along the D and J helices and face each other directly across the heterodimer interface [12] . In these mutants, the formation of disulphide bridges across subunits would require protomers to move closer together than illustrated by the structural model of the GluN1/GluN2A dimer LBD fragment, but would preserve the relative orientation of protomers within the dimer. Similar to Mt1/Mt1 receptors, Mt2/Mt2 receptors produced normally desensitizing currents and DTT strongly potentiated peak current amplitude ( I pk ) and reduced desensitization ( I ss / I pk and τ D ; Fig. 1e ). These results indicate that the observed loss of activity originated from a loss of flexibility across the dimer interface and was not residue-specific. This loss of flexibility did not visibly affect macroscopic desensitization as determined by comparing mutant with Wt whole-cell current traces. Contrary to expectations, restoring flexibility at the dimer interface by treating either mutant with DTT caused currents to desensitize less and with slower kinetics. Next, we used bifunctional crosslinkers of several lengths to test whether receptor activation required intersubunit proximity or just interface flexibility. A disulfonate reagent methanethiosulfonate (MTS)1, which when bound would allow a maximal separation of ~4.7 Å between the engineered cysteines, decreased whole-cell currents recorded from DTT-treated Mt1/Mt1 receptors to the same extent as direct crosslinking (disulphide bond, ~2 Å). MTS reagents with longer linkers (5.7 Å for MTS2 and 7.1 Å for MTS3) prevented activation even more severely ( Fig. 1f ). Consistently, MTS tethering of subunits produced faster desensitizing macroscopic currents. These results are in contrast with the observation that MTS-tethering of subunits within dimers potentiate current amplitudes and reduce desensitization in AMPA receptors [7] . Together they indicate that the dimer interface may have a distinct role in NMDA receptor activation, one that requires both protomer proximity and a flexible interface. To investigate this novel hypothesis, we examined the reaction mechanism of Mt1/Mt1 receptors at the single-molecule level. Crosslinked Mt1/Mt1 receptors open infrequently and briefly We recorded on-cell single-channel currents from Mt1/Mt1 receptors with high agonist concentrations in the recording pipette (1 mM glutamate and 0.1 mM glycine), condition, which causes the receptors to be essentially fully liganded ( n =6). In all records, Mt1/Mt1 channels displayed bursting behaviour, a direct indication that channels entered desensitized states despite covalent tethering of the dimer interface. Furthermore, we observed that overall channel activity was drastically reduced ( Fig. 2a ). The measured open probability ( P o ) of Mt1/Mt1 receptors was ~200-fold lower than that of Wt/Wt receptors. Mean closed time was increased >100-fold and mean open time was reduced fourfold ( Table 1 ). Notably, the large increase in mean closed time reflected entirely longer closures within bursts, while the duration of closures between bursts, which correspond to dwells in desensitized states [13] , were intact (τ D , 3.0±0.4 s for Mt1/Mt1 versus 2.7±0.3 for Wt/Wt, P >0.05, two-tailed Student's t -test) ( Fig. 2b ; Table 1 ). This result represents strong evidence that crosslinked receptors had severely reduced activity due to longer intraburst closures and shorter openings but had intact microscopic desensitization. 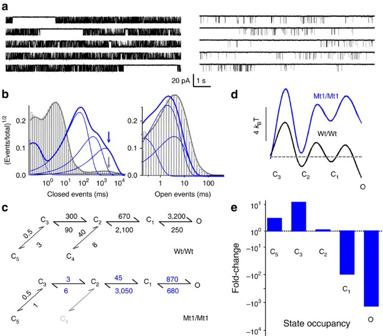Figure 2: Single-molecule activity of NMDA receptors with crosslinked dimers. (a) Continuous traces recorded from on-cell patches containing one Wt/Wt (left) or one Mt1/Mt1 receptor (right). (b) Overlaid event histograms calculated from the records illustrated inafor Wt/Wt (grey) and Mt1/Mt1 (blue) receptors. Arrows point to the longest closed component, which is of similar duration for both receptors. (c) Reaction mechanisms show best-fitting schemes to stationary single-channel activity for Wt/Wt (n=18) and Mt1/Mt1 (n=6) receptors. Transitions into state C4(grey) were not detected for crosslinked receptors. Rate constants (s−1) are given as rounded means of the values estimated from each data set; blue indicatesP<0.05 relative to Wt/Wt (Student'st-test). (d) Relative free-energy profiles calculated from the models incaligned to the first liganded state. (e) Change in fractional state occupancies calculated from the models inc. Figure 2: Single-molecule activity of NMDA receptors with crosslinked dimers. ( a ) Continuous traces recorded from on-cell patches containing one Wt/Wt (left) or one Mt1/Mt1 receptor (right). ( b ) Overlaid event histograms calculated from the records illustrated in a for Wt/Wt (grey) and Mt1/Mt1 (blue) receptors. Arrows point to the longest closed component, which is of similar duration for both receptors. ( c ) Reaction mechanisms show best-fitting schemes to stationary single-channel activity for Wt/Wt ( n =18) and Mt1/Mt1 ( n =6) receptors. Transitions into state C 4 (grey) were not detected for crosslinked receptors. Rate constants (s −1 ) are given as rounded means of the values estimated from each data set; blue indicates P <0.05 relative to Wt/Wt (Student's t -test). ( d ) Relative free-energy profiles calculated from the models in c aligned to the first liganded state. ( e ) Change in fractional state occupancies calculated from the models in c . Full size image Table 1 Single channel parameters of NMDA receptors with mutations at the dimer interface. Full size table We next used statistical analyses of event distributions in combination with kinetic modelling to evaluate the reaction mechanism of crosslinked receptors. Previous work has demonstrated that NMDA receptors activate along a complex pathway consisting of three functional steps: agonist binding, receptor activation, and receptor desensitization [14] , [15] . Activation can be further decomposed into three sequential rearrangements: C 3 →C 2 →C 1 →O, where C 3−1 denote three kinetically distinct preopen states and O represents several linked open states [16] , [17] , [18] , [19] . Desensitization is often depicted as two separate transitions that diverge from the main activation pathway: C 3 -C 5 and C 2 -C 4 , where C 5 represents the main, most stable desensitized state and C 4 represents a minor, less prominent desensitized state [20] , [21] ( Fig. 2c ). We found that Mt1/Mt1 receptors followed a reaction mechanism similar to Wt NMDA receptors; the single difference was the absence of the minor desensitized state C 4 , perhaps due to decreased kinetic resolution in this low-activity mutant. Macroscopic currents simulated with this state model resembled closely the time course of experimentally recorded whole-cell and excised-patch responses from a similar preparation, further reinforcing this model's validity ( Fig. 2c ; Supplementary Figs S2 and S3 ). The model attributes the low P o of crosslinked receptors to substantially slower activation and faster deactivation transitions while clearly demonstrating normal microscopic desensitization ( Fig. 2c ). On the basis of the relative free-energy profile calculated from this model, we propose that NMDA receptors with crosslinked heterodimer interfaces cannot open properly due to higher energy barriers to activation and substantially destabilized open states ( Fig. 2d ). The implication is that when the D1-D1 interfaces of NMDA receptors are frozen in the arrangement described by Furukawa et al . [12] receptors are most likely closed, residing primarily in preopen C 3 and desensitized C 5 conformations ( Fig. 2e ). A flexible dimer interface is required for normal openings Further, we examined the activation mechanism of three NMDA receptor mutants that had free cysteine residues facing the dimer interface: DTT-treated Mt1/Mt1, Mt1/Wt and Wt/Mt1 receptors. On the basis of the available structural data, we reasoned that these receptors would have overall weaker dimer interfaces relative to Wt/Wt receptors due to a two-bond deficit in each LBD dimer: one hydrogen bond and one Van der Waals interaction. On the basis of the marked potentiation of whole-cell Mt1/Mt1 currents by DTT ( Fig. 1b ), we expected that reduced Mt1/Mt1 would generate higher single-channel activity than crosslinked Mt1/Mt1, but we could not anticipate how these activities would compare with Wt/Wt. Indeed, we found that all three receptors investigated, DTT-treated Mt1/Mt1, Mt1/Wt and Wt/Mt1, had substantially higher P o values (>50-fold) than crosslinked Mt1/Mt1; in addition, we were able to determine that their P o values remained substantially lower (<4-fold) than Wt/Wt receptors ( Fig. 3a ; Table 1 ). Remarkably, the absence of a restraining disulphide bond in these mutant receptors resulted in Wt-like openings, a clue that restoring flexibility at the dimer interface may have restored open state stabilities ( Fig. 3b ; Table 1 ). 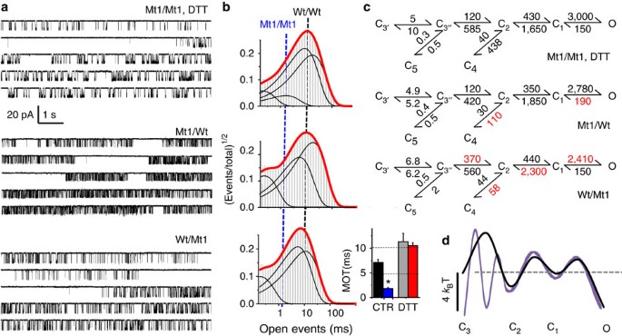Figure 3: Single-molecule activity of NMDAR receptors with destabilized LBD interfaces. (a) Portions of continuous one-channel activity recorded from receptors that have cysteine residues substituted within the hydrophobic cores of ligand binding domain dimers. (b) Open event distributions calculated from the records illustrated ina. Dotted lines show relative position of mean open times calculated for Wt/Wt and Mt1/Mt1 receptors. Bar graph shows summary of mean open times (MOTs) (means±s.e.m.) from Wt/Wt (black, grey) and Mt1/Mt1 (blue, red) receptors in control (CTR) and reducing (DTT) conditions. Asterisk indicatesP<0.05 relative to Wt/Wt (Student'sttest). (c) Reaction mechanisms show best fitting schemes to single channel and macroscopic data in each condition. Rate constants are given in s−1as the rounded mean of fits to six one-channel records; in red are rates that are different (P<0.05, Student'st-test) relative to reduced Mt1/Mt1 receptors. (d) Relative free energy landscapes of the main activation pathway for reduced Mt1/Mt1 (purple) and reduced Wt/Wt (black) receptors were aligned to O state levels, based on equal mean open times. Figure 3: Single-molecule activity of NMDAR receptors with destabilized LBD interfaces. ( a ) Portions of continuous one-channel activity recorded from receptors that have cysteine residues substituted within the hydrophobic cores of ligand binding domain dimers. ( b ) Open event distributions calculated from the records illustrated in a . Dotted lines show relative position of mean open times calculated for Wt/Wt and Mt1/Mt1 receptors. Bar graph shows summary of mean open times (MOTs) (means±s.e.m.) from Wt/Wt (black, grey) and Mt1/Mt1 (blue, red) receptors in control (CTR) and reducing (DTT) conditions. Asterisk indicates P <0.05 relative to Wt/Wt (Student's t test). ( c ) Reaction mechanisms show best fitting schemes to single channel and macroscopic data in each condition. Rate constants are given in s −1 as the rounded mean of fits to six one-channel records; in red are rates that are different ( P <0.05, Student's t -test) relative to reduced Mt1/Mt1 receptors. ( d ) Relative free energy landscapes of the main activation pathway for reduced Mt1/Mt1 (purple) and reduced Wt/Wt (black) receptors were aligned to O state levels, based on equal mean open times. Full size image In contrast to Wt/Wt receptors, event distributions of receptors with cysteine residues facing the dimer interface, revealed six rather than five closed components, an indication that these receptors dwell longer in a closed state that is only briefly populated by Wt/Wt receptors. The scheme illustrated in Figure 3c best described both single channel data and macroscopic responses recorded from these mutants ( Supplementary Figs S2b and S3 ). This scheme postulates that after becoming fully liganded, receptors with reduced Mt1 subunits dwell longer in a preopen state (C 3′ ) before accessing a state (C 3″ ) from which they can either desensitize or continue on the activation pathway. A simple interpretation of this result is that the cysteine residues engineered at the dimer interface divided the collection of equienergetic conformers that make up the aggregate state C 3 of Wt/Wt receptors into two kinetically resolvable states, C 3′ and C 3″ ( Fig. 3d ). Consistent with this interpretation, substitutions that preserved or even enhanced the hydrophobic nature of the buried interface produced close to Wt NMDA receptor activity. In the structure represented in Figure 1a , we substituted only one of the two residues in each interacting pair for a tyrosine residue: GluN1(N521Y) for the N521~L780 pair, or/and GluN2A(E516Y) for the symmetrically related L777~E516 pair. Tyrosine-substituted subunits produced Wt activity when paired with a Wt partner and only mildly (twofold) decreased P o when paired together (GluN1(N521Y) with GluN2A(E516Y) ( Table 1 ; Supplementary Fig. S4 )). The lack of kinetic phenotype for these mutants is remarkable because the homologous mutation in AMPA receptors, GluA2 (L483Y), produces largely non-desensitizing receptors [7] , [22] . We conclude that introducing an aromatic (tyrosine) but not a polar residue (cysteine) allows rearrangements at the heterodimer interface without delay or interruption, and that this structural plasticity is required for proper receptor activation. However, in contrast to non-NMDA receptors, neither substitution affects NMDA receptor desensitization. In AMPA- and kainate-type glutamate receptors, the physical separation of subunits within LBDs leads to functional desensitization and this can be prevented by bracing the dimer interface with covalent links across subunits [5] , [6] , [7] , [10] . On the basis of the substantial structural homology demonstrated for glutamate receptor classes the current assumption is that the dimer interface serves a similar function in all glutamate-gated channels, including NMDA receptors. To test this hypothesis we investigated how perturbing contacts between GluN1 and GluN2A subunits in the ligand-binding domains of NMDA receptors influenced the receptor's activation mechanism. We chose to examine substitutions that were previously demonstrated to have significant effects on the macroscopic behaviours of AMPA, kainate and NMDA receptors. Further, we used one-channel current recordings, kinetic analyses and state modelling to examine NMDA receptors whose heterodimers were reinforced with disulphide bridges across the D1-D1 interface or had free cysteine or tyrosine residues facing the intersubunit boundary. Disulphide bridges between LBD protomers prevent AMPA [7] , [10] and kainate [5] , [10] receptor desensitization and render NMDA receptors insensitive to allosteric inhibition [11] . We found that NMDA receptors whose dimer interfaces were locked with disulphide crosslinks in the arrangement described by Furukawa et al . [12] produced normally desensitizing currents, whereas reducing the disulphide bonds increased the macroscopic current and reduced its desensitization ( Fig. 1 ). These results reveal that the strength of contacts at dimer interfaces within LBDs have opposite effects on the shape of the macroscopic currents recorded from NMDA and non-NMDA receptors. At central excitatory synapses the shape of the postsynaptic current results from the combined action of NMDA and non-NMDA classes of glutamate receptors. Each class generates currents with distinct temporal profiles: non-NMDA receptors open and desensitize within milliseconds, whereas NMDA receptors do so much slower, within tens and hundreds of milliseconds, respectively [1] . The characteristic time course of the macroscopic response is rooted in unique reaction mechanisms. Importantly, non-NMDA receptors can open one subunit at a time, indicative of a largely subunit-independent gating mechanism, whereas NMDA receptor subunits are highly coupled during activation. Despite these fundamental differences in kinetics and reaction mechanisms, glutamate receptors share substantial sequence homology and are similar in overall structure [1] , [23] , [24] . At present, extensive structural data support a conserved mechanism for agonist-induced opening of glutamate-gated channels: upon binding, glutamate changes the shape of the LBD in each subunit and this movement is transmitted to adjoining pore-forming helices as long as the LBD dimer remains intact [1] , [2] , [4] . Similarly, strong evidence exists in support of a common desensitization mechanism for AMPA and kainate receptors: the tension resulting from glutamate-induced change in the shape of the LBD in each subunit can cause subunits within the LBD dimers to separate and allows the pore to close while glutamate is still bound [6] , [7] , [8] , [10] . In this context, our results, which clearly show that NMDA receptors with covalently locked dimers desensitize normally, strongly support the assertion that NMDA and non-NMDA receptors have distinct desensitization mechanisms. This is consistent with the marked difference in intersubunit coupling during gating for these receptor types and points to a key role for intersubunit contacts in the divergent reaction mechanisms of structurally similar glutamate-gated channels. The reaction mechanism of NMDA receptor is known in sufficient detail to allow accurate attribution of macroscopic current features such as amplitude and decay time course to microscopic kinetic transitions inferred from the single-channel record, a task not yet possible for non-NMDA receptors. We examined the reaction mechanism of crosslinked NMDA receptors and concluded that indeed receptors with covalently joined subunits had intact microscopic desensitization but their activation was deeply impaired: they had 200-fold lower open probabilities due to increased barriers to activation and unstable open states ( Fig. 2 ). Reducing the disulphide bonds restored open state stabilities but not the height of the activation barriers, which retained receptors in early preopen conformations ( Fig. 3 ). These results led us to hypothesize that in contrast to non-NMDA receptors, a frangible intersubunit interface within the LBDs of NMDA receptors is necessary for activation rather than desensitization. However, simply increasing dimer separation by tethering subunits at fixed lengths with MTS reagents failed to reproduce the activity seen in reducing conditions ( Fig. 1f ), an indication that flexibility at the dimer interface as well as intersubunit proximity are required for effective channel opening. On the basis of these results, we conclude that NMDA receptor activation, but not desensitization, requires rearrangements at the dimer interface described by Furukawa et al . [12] , which likely represents the ligand-binding unit of a closed receptor, an atomic arrangement adopted early in the activation sequence. Taken together, our results demonstrate that changes in the relative positions of residues facing the dimer interface are integral to the activation sequence of NMDA receptors and demonstrate fundamental differences in the activation mechanism of glutamate receptor classes. Molecular biology Plasmids expressing GluN1-1a, GluN2A and GFP were transfected into HEK 293 cells as described in detail previously [20] . Cysteine or tyrosine substitutions were obtained with standard molecular biology procedures and were verified by full-insert sequencing. Macroscopic current recordings and analyses Macroscopic NMDA receptor currents were recorded with the excised-patch or the whole-cell patch clamp techniques where intracellular solutions contained: 135 mM CsF, 33 mM CsOH, 2 mM MgCl 2 , 1 mM CaCl 2 , 10 mM HEPES, 11 mM EGTA, adjusted to pH 7.4 (CsOH) and the holding potential was −70 mV. All extracellular solutions contained: 150 mM NaCl, 2.5 mM KCl, 0.5 mM CaCl 2 , 0.01 mM EDTA and 10 mM HEPBS adjusted to pH 8.0 (NaOH) plus 0.1 mM Gly. Currents were elicited by switching the cell or excised patch into solutions containing Glu (1 mM) [20] , [25] . When specified, DTT (10 mM) or hydrogen peroxide (H 2 O 2 ) (0.5%) was also included. Bifunctional crosslinkers (Toronto Research Chemicals) were prepared from dimethylformamide stocks to 0.5 mM final concentration. Decay time course (τ D ) was evaluated by fits to single-exponential function; steadystate to peak current ratio ( I ss / I pk ) was calculated in pClamp 10.2 (Molecular Devices). Single-channel current recordings and analyses Activity from individual NMDA receptors was recorded using the cell-attached patch-clamp technique with extracellular solutions that contained 150 mM NaCl, 2.5 mM KCl, 10 mM HEPBS, 1 mM EDTA, 1 mM Glu, 0.1 mM Gly adjusted to pH 8 (NaOH), and applying +100 mV through the recording electrode. Currents were analog filtered at 10 kHz and digitally sampled at 40 kHz directly into digital files using the QUB software ( www.qub.buffalo.edu ). Only records originating from one-channel patches were kept and used for analyses [20] , [26] . Idealization, modelling and simulations were carried out in QUB with a 0.15-ms dead time [27] . Simulations Macroscopic responses were calculated as time-dependent occupancies of open states from the models obtained in this study after appending glutamate-binding steps, as previously described [19] , [25] , [28] , [29] . All channels were started in the resting state and glutamate pulses were simulated as instantaneous steps into 1-mM Glu. For each condition, the simulated traces were analysed to extract desensitization time constants (τ D ) and I ss / I pk ratios as for experimentally recorded traces. How to cite this article: Borschel, W. F. et al . NMDA receptor activation requires remodelling of intersubunit contacts within ligand-binding heterodimers. Nat. Commun. 2:498 doi: 10.1038/ncomms1512 (2011).